Reply to: Reconciling differences in impact of molecular subtyping on response to cisplatin-based chemotherapy 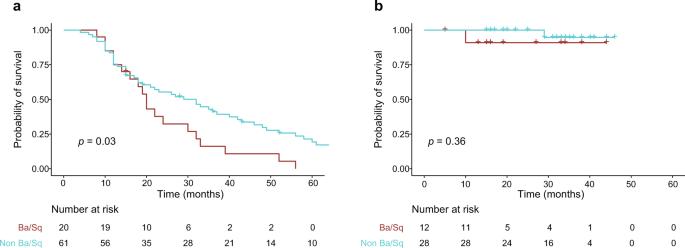Fig. 1: Kaplan–Meier survival analysis stratified by gene expression subtype. Probability of overall survival for patients treated with first-line chemotherapy (a) or NAC (b) with and without Ba/Sq gene expression subtype.Pvalues were calculated using a log-rank test for comparing survival curves. Source data are provided as a Source data file. Information regarding patients, tissue samples, nucleotide extraction procedure, and RNA-sequencing (RNA-seq) is provided in ref. [9] . RNA-seq data were available for 121 patients (NAC: n = 40, first-line n = 81). Gene expression consensus subtypes were called as described in ref. [9] Cumulative survival analysis was performed using the Kaplan–Meier method, and the log-rank test was used to compare the curves (R packages survminer and survival). OS was defined as time from MIBC diagnosis to death or end of follow-up. Reporting summary Further information on research design is available in the Nature Research Reporting Summary linked to this article.